Lysosomal NEU1 deficiency affects amyloid precursor protein levels and amyloid-β secretion via deregulated lysosomal exocytosis Alzheimer’s disease (AD) belongs to a category of adult neurodegenerative conditions, which are associated with intracellular and extracellular accumulation of neurotoxic protein aggregates. Understanding how these aggregates are formed, secreted and propagated by neurons has been the subject of intensive research, but so far no preventive or curative therapy for AD is available, and clinical trials have been largely unsuccessful. Here we show that deficiency of the lysosomal sialidase NEU1 leads to the spontaneous occurrence of an AD-like amyloidogenic process in mice. This involves two consecutive events linked to NEU1 loss-of-function—accumulation and amyloidogenic processing of an oversialylated amyloid precursor protein in lysosomes, and extracellular release of Aβ peptides by excessive lysosomal exocytosis. Furthermore, cerebral injection of NEU1 in an established AD mouse model substantially reduces β-amyloid plaques. Our findings identify an additional pathway for the secretion of Aβ and define NEU1 as a potential therapeutic molecule for AD. Amyloidoses comprise a group of diseases characterized by the abnormal deposition of insoluble fibrillar proteins, called amyloid deposits, in different organs, including the brain [1] . These deposits are usually the result of increased synthesis or altered degradation of specific proteins or protein fragments. Amyloid deposition in the brain is the hallmark of Alzheimer’s disease (AD), the most prevalent, age-related neurodegenerative condition worldwide, which is associated with progressive decline of cognitive functions and dementia [2] . Although the precise mechanisms leading to AD pathology are not yet fully understood, it is well established that the two types of protein aggregates accumulating in AD brains are primarily composed of proteolytic fragments of the amyloid precursor protein (APP) and τ-containing neurofibrillary tangles. Aberrant processing of APP by the β-secretase BACE1 (β-site APP-cleaving enzyme 1) generates an amyloidogenic APP carboxy-terminal fragment (CTF), which is further cleaved by the presenilin-containing γ-secretase complex into two main amyloid β-peptide isoforms (Aβ): Aβ-40 and Aβ-42 (refs 3 , 4 , 5 ). Aβ-42 is considered the most toxic peptide, which in vitro assembles into fibrils at micromolar concentrations and at acidic pH, and functions in vivo as seeding point for the deposition of amyloid into senile plaques [6] , [7] , [8] . Although most of the Aβ is found extracellularly, it is now accepted that it may also reside in neurons [9] , [10] , [11] . This intracellular pool may be linked to extracellular Aβ, because an inverse relationship between plaque numbers and Aβ intraneuronal immunoreactivity has been demonstrated [10] . These findings suggest that the intracellular accumulation of Aβ represents an early event in AD aetiology, preceding the deposition of the extracellular pool [9] , [11] . It is still unclear, however, how this intracellular Aβ is deposited outside the cells and how it aggregates into plaques. It has been proposed that Aβ, similar to other toxic proteins, can ‘spread’ from one cell to another via prion-like mechanisms of transmission, including passive release/membrane rupture, cell to cell nanotubes and exocytosis [12] , [13] . Indeed, it has been shown that intracellular Aβ oligomers can be transferred from neuron to neuron via direct contacts [14] , and APP, CTF and Aβ have been found in multivesicular bodies and released in association with exosomes [15] , [16] , [17] , [18] . These recent observations raise the possibility that intracellular Aβ can be released by these or other, as yet unknown, regulated exocytic processes. The extracellular Aβ may then be recaptured by an endocytic mechanism by neighbouring or distant neurons, thereby propagating the transmission of the toxic peptide. In fact, changes in the morphology and function of the endosomal system have been described as the earliest biochemical alterations seen in AD brains [11] , [19] , [20] , [21] . In addition, the findings of reduced autophagic clearance [22] and accumulation of lysosomal cathepsins in the amyloid plaques [23] , [24] , [25] directly implicate the lysosomal compartment in the development and progression of AD. The importance of a fully functional lysosomal system in neural cell homeostasis is well recognized in the large group of neurodegenerative lysosomal storage diseases (LSDs). These primarily pediatric disorders often display signs of premature cellular aging [26] . Therefore, they may represent ideal models to identify basic mechanisms of central nervous system pathogenesis and provide insight into more common, adult neurodegenerative conditions. This has been recently highlighted by the discovery of a genetic association between Parkinsonism and Gaucher disease, caused by mutations in the glucocerebrosidase gene, GBA1 (refs 27 , 28 ). Parkinson’s disease patients have an increased rate of GBA1 mutations, defining lysosomal GBA1 as the most common risk factor for the development of this disease. We now provide evidence, in mice, of another link between age-related neurodegeneration and lysosomal dysfunction, by showing that deficiency of the lysosomal sialidase NEU1 (neuraminidase 1) in the LSD sialidosis is at the basis of an amyloidogenic process reminiscent of AD. In normal conditions, NEU1 initiates the catabolism of sialoglyconjugates by removing their terminal sialic acids [29] . The enzyme depends on its interaction with the auxiliary protein, protective protein/cathepsin A (PPCA), for its compartmentalization in lysosomes and catalytic activation [30] . Aside from its canonical degradative function, NEU1 regulates the physiological process of lysosomal exocytosis by controlling the sialic acid content of the lysosomal-associated membrane protein-1, LAMP1 (ref. 31 ). Lysosomal exocytosis is a calcium-regulated process that entails the recruitment along the cytoskeletal network of a pool of lysosomes destined to dock at the plasma membrane (PM); this step is mediated by LAMP1. Docked lysosomes then fuse their limiting membrane with the PM in response to calcium influx and release their luminal content extracellularly. Lysosomal exocytosis has a role in the regulated secretion of lysosomal contents in specialized cells [32] , and in the replenishment and repair of the PM in virtually all cell types [31] , [33] . In the absence of NEU1, oversialylated LAMP1 marks an increased number of lysosomes poised to dock at the PM and engage in lysosomal exocytosis. The end result is the exacerbated release of lysosomal contents, which abnormally remodels the extracellular matrix and changes its composition, along with that of the PM. Here we investigate the role of NEU1 and lysosomal exocytosis in the amyloidogenic process found in the brain of the Neu1 −/− mice, the only model of excessive lysosomal exocytosis. We show that this process begins with the accumulation in endolysosomes of an oversialylated APP, a newly identified substrate of NEU1. Endolysosomal APP is then proteolytically cleaved to generate Aβ, which is ultimately released extracellularly by excessive lysosomal exocytosis. Remarkably, intracranial injection of NEU1 in the AD model 5XFAD reduces the numbers of amyloid plaques and the levels of amyloid peptides. Thus, NEU1 may represent a risk factor for the development of AD-like amyloidosis and, in this respect, could be explored as a therapeutic approach for AD. Excessive lysosomal exocytosis in Neu1 −/− neural cells Neu1 −/− mice have profound systemic and neurological abnormalities, are smaller in size than their wild-type (WT) littermates and have a shortened lifespan (~5 months). At a late stage of the disease, they appear weak and debilitated, and suffer from dyspnoea, oedema, gait abnormalities and tremor [34] , [35] . By mapping Neu1 expression in the WT mouse brain, we found that the enzyme was distributed evenly throughout the parenchyma ( Supplementary Figs S1 and S2 ), but was particularly abundant in the hippocampus ( Fig. 1a ). In the Neu1 −/− brain, deficiency of the enzyme was accompanied by increased levels of Lamp1, whose expression is normally low in the WT brain ( Fig. 1c ). In addition, Lamp1 accumulated in an oversialylated state ( Fig. 1b ). Although Lamp1 has been found to be upregulated in other LSDs [36] , [37] due to expansion of the lysosomal compartment, in the context of a Neu1 deficiency upregulation of the protein coupled to its oversialylation results in increased lysosomal exocytosis [31] , [38] . Thus, we tested the extent of lysosomal exocytosis in primary neurospheres, by measuring as marker of this process the activity of the lysosomal β-hexosaminidase (β-hex) [33] , [39] in the culture medium. These cells were isolated from pups obtained by crossing WT or Neu1 −/− mice with Arf −/− mice [40] , to improve their self-renewal and culturing time [41] , [42] . Neurospheres from WT/Arf −/− ( WT Arf ) and Neu1 −/− /Arf −/− ( Neu1 −/−/Arf ) had similar cell composition ( Supplementary Fig. S3a ), but β-hex activity was substantially increased only in the medium of the Neu1 −/−/Arf neurospheres but not in their cell pellets ( Fig. 1d and Supplementary Fig S3b ). Thus, excessive lysosomal exocytosis occurs in the deficient cells. In contrast, β-hex activity measured in the medium of neurospheres isolated from β-galactosidase-deficient mice, a model of the LSD GM1 gangliosidosis [43] , was in the normal range ( Fig. 1d ), indicating that exacerbated lysosomal exocytosis is linked to Neu1 deficiency. To determine which cell type in the neurosphere cultures was more exocytic, we assayed for lysosomal exocytosis WT and Neu1 −/− primary astrocytes and hippocampal neurons differentiated from neurospheres [44] ( Fig. 1e and Supplementary Fig. S3c ). The activity of β-hex was comparable in the medium of the astrocyte cultures ( Supplementary Fig. S3d ), whereas it was increased in the medium of Neu1 −/− neurons ( Fig. 1f ), defining this population of cells as the most exocytic. Thus, Neu1 deficiency in neurons enhances their lysosomal exocytosis potential. 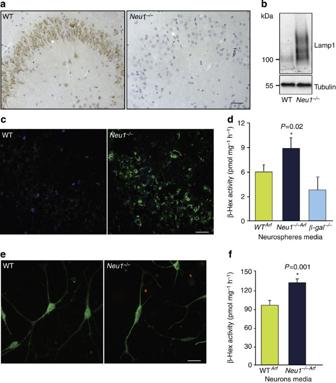Figure 1: Altered expression of Lamp1 in the brain ofNeu1−/−mice. (a) Neu1 expression is high in the CA3 region of the WT hippocampus. (b) Oversialylation of Lamp1 shown on immunoblots of WT andNeu1−/−hippocampal lysates probed with the indicated antibody. (c) Loss of Neu1 is accompanied by accumulation of Lamp1. (d) Extent of lysosomal exocytosis measured as β-hex enzyme activity in the culture medium of neurospheres.Neu1−/−/Arfhippocampal neurospheres have enhanced lysosomal exocytosis. (e) Representative picture ofWTArfandNeu1−/−/Arfhippocampal neurons stained with β-III tubulin (green) and glial fibrillary acidic protein (GFAP; red). (f)Neu1−/−/Arfhippocampal neurons have enhanced lysosomal exocytosis as assessed by β-hex enzyme activity measured in the culture medium. Asterisks indicate statistically significant results, as determined by the Student’st-test. Data are represented as mean±s.d. (error bars);n=3. Mice used for histological analyses were 5 months of age. Scale bars, 20 μm. Figure 1: Altered expression of Lamp1 in the brain of Neu1 −/− mice. ( a ) Neu1 expression is high in the CA3 region of the WT hippocampus. ( b ) Oversialylation of Lamp1 shown on immunoblots of WT and Neu1 −/− hippocampal lysates probed with the indicated antibody. ( c ) Loss of Neu1 is accompanied by accumulation of Lamp1. ( d ) Extent of lysosomal exocytosis measured as β-hex enzyme activity in the culture medium of neurospheres. Neu1 −/−/Arf hippocampal neurospheres have enhanced lysosomal exocytosis. ( e ) Representative picture of WT Arf and Neu1 −/−/Arf hippocampal neurons stained with β-III tubulin (green) and glial fibrillary acidic protein (GFAP; red). ( f ) Neu1 −/−/Arf hippocampal neurons have enhanced lysosomal exocytosis as assessed by β-hex enzyme activity measured in the culture medium. Asterisks indicate statistically significant results, as determined by the Student’s t- test. Data are represented as mean±s.d. (error bars); n =3. Mice used for histological analyses were 5 months of age. Scale bars, 20 μm. Full size image Neu1 deficiency leads to AD-like pathology Increased exocytosis of lysosomal contents from neurons could impact on the architecture and composition of the brain parenchyma. In fact, histopathological examination of the Neu1 −/− brain identified numerous abnormal eosinophilic bodies, primarily clustered in the CA3 region of the hippocampus ( Fig. 2a ) and the fimbria. These bodies were heterogeneous in size and shape, and mostly contained amorphous, granular, proteinaceous material that resembled amyloid. They were visualized throughout the CA3 region and, to some extent, in the cortex, after systemic, in vivo injection of Neu1 −/− mice with the Congo red/Chrysamine-G fluorescent derivative Methoxy-X04, which has been shown to bind with high affinity to amyloid fibrils [45] ( Fig. 2b,c ). Furthermore, ultrastructural examination of the Neu1 −/− hippocampal region identified numerous swollen dystrophic neurites ( Supplementary Fig. S4 ), a feature also associated with amyloid plaques. Combined, these pathological changes downstream of Neu1 deficiency were reminiscent of those seen in several neurological amyloidoses, including early-stage AD [46] . 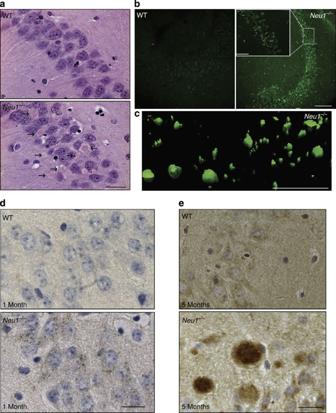Figure 2: Pathologic abnormalities in theNeu1−/−hippocampus. (a) haematoxylin and eosin staining demonstrated numerous eosinophilic bodies (arrows) in the CA3 region of theNeu1−/−brain (mice 5 months of age). Scale bar, 20 μm. (b) Methoxy-XO-4-stained amyloid deposits inNeu1−/−hippocampus. Scale bars, 100 μm (mice 5 months of age; scale bar, 50 μm for zoom in). (c)Z-stacks obtained from confocal images ofNeu1−/−. Methoxy-XO4+ amyloid deposits were used to build a three-dimensional surface rendering. Scale, bar 250 μm. (d) In theNeu1−/−hippocampus, APP starts to accumulate intracellularly as early as 1 month of age, as revealed by IHC analysis with anti-APP N-terminal antibody (brown). (e) Amyloid deposits in 5-month-oldNeu1−/−brain stained positive for APP (N-terminal antibody). (d,e) Scale bars, 20 μm. Figure 2: Pathologic abnormalities in the Neu1 −/− hippocampus. ( a ) haematoxylin and eosin staining demonstrated numerous eosinophilic bodies (arrows) in the CA3 region of the Neu1 −/− brain (mice 5 months of age). Scale bar, 20 μm. ( b ) Methoxy-XO-4-stained amyloid deposits in Neu1 −/− hippocampus. Scale bars, 100 μm (mice 5 months of age; scale bar, 50 μm for zoom in). ( c ) Z -stacks obtained from confocal images of Neu1 −/− . Methoxy-XO4+ amyloid deposits were used to build a three-dimensional surface rendering. Scale, bar 250 μm. ( d ) In the Neu1 −/− hippocampus, APP starts to accumulate intracellularly as early as 1 month of age, as revealed by IHC analysis with anti-APP N-terminal antibody (brown). ( e ) Amyloid deposits in 5-month-old Neu1 −/− brain stained positive for APP (N-terminal antibody). ( d , e ) Scale bars, 20 μm. Full size image We therefore asked whether the amyloid bodies spontaneously arising in Neu1 −/− brains shared features with Alzheimer β-amyloid. To address this point, we performed a series of immunostainings of brain sections, using antibodies against full-length APP (amino-terminal antibody). We found that APP accumulated in the Neu1 −/− CA3 hippocampal neurons as early as 1 month of age and was resolved in discrete intracellular puncta ( Fig. 2d ). As the animals aged, APP + bodies increasingly formed ( Fig. 2e ) and were most prominent towards the end of their lifespan. At this time point, the majority of these bodies were also immunoreactive for ubiquitin and neurofilaments, indicating that Neu1 −/− hippocampal neurons underwent extensive cytoskeletal remodelling and showed impaired intracellular trafficking ( Supplementary Fig. S5a,b ). Accumulation of APP was also assessed by quantitative analysis of band intensity on immunoblots of Neu1 −/− hippocampal lysates ( Fig. 3a,b ). The presence of amyloid deposits and accumulated APP in the Neu1 −/− mice support the idea that NEU1 deficiency may predispose to an AD-like phenotype. 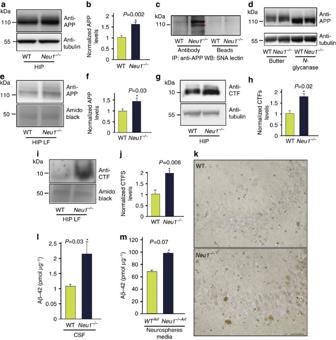Figure 3: APP is a natural substrate of Neu1 and is abnormally processed inNeu1−/−lysosomes. (a,b) APP levels are increased inNeu1−/−total hippocampal (HIP) lysates as demonstrated by immunoblots (a) and by densitometric analysis (b). (c) APP was immunoprecipitated from WT andNeu1−/−HIP and probed on blots withSanbucus nigralectin (SNA). (d) Equal amounts of HIP lysates were treated withN-glycanase, sialidase and probed on blots with anti-APP N-terminal antibody. (e) Immunoblots of WT andNeu1−/−HIP-enriched LF shows APP accumulation in theNeu1−/−samples. (f) Quantification ofe. (g,i) β-CTF levels are increased inNeu1−/−HIP lysates andNeu1−/−HIP-enriched LF, respectively. (h,j) Quantification ofgandi. (k) Representative Aβ peptide staining in WT andNeu1−/−brain sections shows immunoreactivity only inNeu1−/−specimens (mouse-specific pan-Aβ-antibody used on 5-month-old brain sections). Scale bar, 20 μm. (l,m) Levels of mouse Aβ42 assayed in the cerebrospinal fluid (CSF) and in the culture medium of neurospheres, respectively. Normalized APP and CTFs refer to the ratio of WT versusNeu1−/−bands. These were calculated by densitometric analysis of single bands on immunoblots probed with anti-APP or β-CTF antibodies, and amido black bands and anti-tubulin in WT andNeu1−/−samples. Red asterisks incdenote oversialylated bands. Asterisks on graphic bars indicate statistically significant results, as determined by the Student’st-test. Data are represented as the mean±s.d. (error bars);n=3. Figure 3: APP is a natural substrate of Neu1 and is abnormally processed in Neu1 −/− lysosomes. ( a , b ) APP levels are increased in Neu1 −/− total hippocampal (HIP) lysates as demonstrated by immunoblots ( a ) and by densitometric analysis ( b ). ( c ) APP was immunoprecipitated from WT and Neu1 −/− HIP and probed on blots with Sanbucus nigra lectin (SNA). ( d ) Equal amounts of HIP lysates were treated with N -glycanase, sialidase and probed on blots with anti-APP N-terminal antibody. ( e ) Immunoblots of WT and Neu1 −/− HIP-enriched LF shows APP accumulation in the Neu1 −/− samples. ( f ) Quantification of e . ( g , i ) β-CTF levels are increased in Neu1 −/− HIP lysates and Neu1 −/− HIP-enriched LF, respectively. ( h , j ) Quantification of g and i . ( k ) Representative Aβ peptide staining in WT and Neu1 −/− brain sections shows immunoreactivity only in Neu1 −/− specimens (mouse-specific pan-Aβ-antibody used on 5-month-old brain sections). Scale bar, 20 μm. ( l , m ) Levels of mouse Aβ42 assayed in the cerebrospinal fluid (CSF) and in the culture medium of neurospheres, respectively. Normalized APP and CTFs refer to the ratio of WT versus Neu1 −/− bands. These were calculated by densitometric analysis of single bands on immunoblots probed with anti-APP or β-CTF antibodies, and amido black bands and anti-tubulin in WT and Neu1 −/− samples. Red asterisks in c denote oversialylated bands. Asterisks on graphic bars indicate statistically significant results, as determined by the Student’s t- test. Data are represented as the mean±s.d. (error bars); n =3. Full size image APP is a natural substrate of NEU1 Given that APP is a glycosylated and sialylated integral membrane protein that was shown to localize in purified lysosomes [47] , and that changes in its glycan composition can cause spurious proteolytic cleavage of the protein, leading to increased formation of Aβ [48] , we thought of testing whether APP could be processed by Neu1 in lysosomes. For this purpose, we first analysed the sialylation status of APP by probing immunoblots of Neu1 −/− hippocampal lysates with Sambucus nigra lectin, which binds with high affinity to α-2,6-linked sialic acids. The results showed that in the absence of Neu1, APP had increased levels of sialic acids compared with the WT protein ( Fig. 3c ). In vitro enzymatic removal of all N -glycans released a core APP protein that was identical in size in the Neu1 −/− and WT samples, indicating that the changes in APP levels in the Neu1 −/− brain were due to the impaired removal of its sialic acids ( Fig. 3d ). We next purified lysosomes from Neu1 −/− and WT hippocampi through a density gradient. Those fractions with the highest lysosomal acid phosphatase activity ( Supplementary Fig. S6 ) were used for biochemical analyses; indeed, APP was increased in pure lysosomal fractions (LFs) from Neu1 −/− hippocampi ( Fig. 3e,f ). Hence, APP is a bona fide substrate of NEU1 and remains oversialylated in the absence of this enzyme activity. The lack of processing of APP’s glycan chains may lengthen its half-life and explain its accumulation in lysosomes. A determining step in the amyloidogenic processing of APP is the generation of CTFs, which are subsequently cleaved into Aβ [3] . We thought to ascertain the extent of CTF generated in the Neu1 −/− hippocampus as predictive measure of abnormal Aβ processing. CTF levels were substantially elevated in both total hippocampal lysates and LFs isolated from the Neu1 −/− brains ( Fig. 3g–j ) compared with those in WT samples. The increased CTF in Neu1 −/− LFs were proteolytically cleaved into Aβ, because we were able to detect endogenous Aβ peptides in Neu1 −/− brain sections, probed with a rodent-specific pan-anti-Aβ antibody, but not in WT sections ( Fig. 3k ). These results prompted us to test for the presence of Aβ42 in the cerebrospinal fluid isolated from WT and Neu1 −/− mice, as well as in the culture media of Neu1 Arf and Neu1 −/−/Arf neurospheres. In both sets of Neu1 −/− samples, we measured substantially increased levels of this peptide ( Fig. 3l,m ). These results suggest that accumulated APP and CTF are processed into Aβ42 in the lysosomal compartment. Excessive lysosomal exocytosis promotes Aβ peptide release Given that loss of Neu1 is associated with increased lysosomal exocytosis, we argued that this process could mediate the extracellular release of lysosomally generated Aβ42 from lysosomes. To test this, we cultured WT Arf and Neu1 −/−/Arf neurospheres in the presence of a human, TAMRA-conjugated, fluorescent Aβ42 (T-Aβ) [8] . T-Aβ was similarly taken up by both WT and Neu1 −/− cell populations and routed to late endosomes/lysosomes ( Fig. 4a ). This fraction of the internalized peptide was then trafficked from the endosomes/lysosomes to the PM, as determined by live imaging of lysotracker-labelled lysosomes with total internal reflection microscopy (TIRFM; Fig. 4b ). This technique allows the visualization of fluorescently labelled organelles in the evanescent field near the cell surface [31] . Quantification of the number of lysotracker + organelles proximal to the PM ( Fig. 4c ) showed that Neu1 −/−/Arf cells had substantially more T-Aβ-containing lysosomes clustered at the PM than did WT Arf cells ( Fig. 4d ). Moreover, when neurospheres were maintained in T-Aβ-free medium for 24 h after exposure to the peptide, we could recover more T-Aβ fluorescence exocytosed from the Neu1 −/−/Arf cells than from the WT Arf cells ( Fig. 4e ). To further confirm that the Aβ peptide was released from Neu1 −/− cells by lysosomal exocytosis, we tested whether induction/inhibition of this process would affect the amount of Aβ peptide released in the medium. WT Arf and Neu1 −/−/Arf neurospheres were cultured in the presence of T-Aβ for 24 h; cells were then treated with the calcium ionophore calcimycin, which enhances lysosomal exocytosis by promoting the calcium-dependent fusion of lysosomes docked at the PM [39] . We found that the medium from calcimycin-treated Neu1 −/−/Arf neurospheres had higher levels of β-hex activity than that from treated WT cells ( Fig. 4f ). This was paralleled by substantially increased levels of Aβ-42 peptide in the calcimycin-treated Neu1 −/− samples ( Fig. 4g ). Most importantly, Neu1 −/− cells maintained in calcium-free medium (+EGTA) before the assays to inhibit lysosomal exocytosis had normal levels of both β-hex and Aβ peptide measured in their culture medium ( Fig. 4f,g ). Thus, in the absence of Neu1, Aβ is abnormally exocytosed by lysosomes, a finding that identifies lysosomal exocytosis as an additional mechanism for the extracellular release of this peptide. 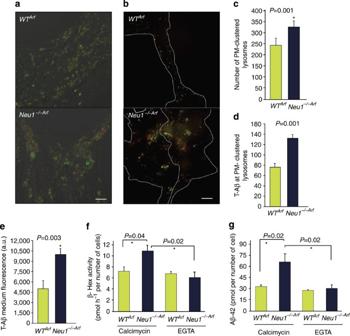Figure 4: Neu1 deficiency and consequent exacerbated lysosomal exocytosis promotes Aβ peptide release. (a) Neurospheres isolated fromWTArfandNeu1−/−/Arfbrains were maintained in culture in the presence of exogenous T-Aβ42 for 24 h and then imaged with confocal microscopy. T-Aβ42 fluorescence (red fluorescence of TAMRA-Aβ42) co-localized with lysotracker (green), marker of endosomes/lysosomes. (b) TIRF analysis shows thatNeu1−/−/Arfhippocampal neurospheres have enhanced T-Aβ levels in PM-docked lysosomes (lysostracker green). (c) Quantification of PM-docked lysosomes shows an increased number of clustered organelles at the PM ofNeu1−/−/Arfcells. (d) Quantification of T-Aβ levels present in PM-docked lysosomes shows higher amounts of T-Aβ inNeu1−/−/Arfcells than in WT samples. (e) TAMRA fluorescence was assayed in neurospheres’ culture medium as an indicator of the levels of T-Aβ released by lysosomal exocytosis. (f,g) Extent of lysosomal exocytosis measured as β-hex enzyme activity and human Aβ-42 assayed in the culture medium ofWTArfandNeu1−/−/Arfneurospheres treated with the calcium ionophore calcimycin in the presence or absence of EGTA, which effectively blocks the lysosomal exocytosis. Asterisks on graphic bars indicate statistically significant results, as determined by the Student’st-test. Data are represented as the mean±s.d. (error bars);n=3. (a,b) Scale bars, 20 μm. Figure 4: Neu1 deficiency and consequent exacerbated lysosomal exocytosis promotes Aβ peptide release. ( a ) Neurospheres isolated from WT Arf and Neu1 −/−/Arf brains were maintained in culture in the presence of exogenous T-Aβ42 for 24 h and then imaged with confocal microscopy. T-Aβ42 fluorescence (red fluorescence of TAMRA-Aβ42) co-localized with lysotracker (green), marker of endosomes/lysosomes. ( b ) TIRF analysis shows that Neu1 −/−/Arf hippocampal neurospheres have enhanced T-Aβ levels in PM-docked lysosomes (lysostracker green). ( c ) Quantification of PM-docked lysosomes shows an increased number of clustered organelles at the PM of Neu1 −/−/Arf cells. ( d ) Quantification of T-Aβ levels present in PM-docked lysosomes shows higher amounts of T-Aβ in Neu1 −/−/Arf cells than in WT samples. ( e ) TAMRA fluorescence was assayed in neurospheres’ culture medium as an indicator of the levels of T-Aβ released by lysosomal exocytosis. ( f , g ) Extent of lysosomal exocytosis measured as β-hex enzyme activity and human Aβ-42 assayed in the culture medium of WT Arf and Neu1 −/−/Arf neurospheres treated with the calcium ionophore calcimycin in the presence or absence of EGTA, which effectively blocks the lysosomal exocytosis. Asterisks on graphic bars indicate statistically significant results, as determined by the Student’s t- test. Data are represented as the mean±s.d. (error bars); n =3. ( a , b ) Scale bars, 20 μm. Full size image NEU1 ablation affects plaque formation in 5XFAD mice Our results so far point to a Neu1-dependent AD-like amyloidogenic process arising spontaneously in the Neu1 −/− mice. To further ascertain whether Neu1 deficiency could exacerbate an existing amyloidogenic process, we crossed the Neu1 −/− mice with a well-characterized model of early-onset familial AD, the 5XFAD mice [49] . These mice overexpress human APP and presenilin-1, both harbouring mutations found in AD patients. Expression of the transgenes is under the control of the neural-specific elements of the mouse Thy1 promoter. In 5XFAD mice, intraneuronal Aβ-42 accumulation starts at 6 weeks of age just before amyloid deposition, which begins in the subiculum of the hippocampus at 2 months and propagates throughout the brain in older mice [49] . We first assessed the effects of Neu1 ablation in the double mutant mice ( 5XFAD / Neu1 −/− ) by recording their ambulatory activity in an open space. Both the double mutants and the Neu1 −/− mice showed similar walking pattern abnormalities and limited exploratory capacity ( Supplementary Movies 1–4 ). We next demonstrated that APP was present in higher amounts in hippocampal lysates from 5XFAD / Neu1 −/− double mutants than in those from 5XFAD mice ( Fig. 5a,b ). Remarkably, APP levels in Neu1 −/− lysates were comparable to those in 5XFAD ( Fig. 5a ). Accumulation of APP was paralleled by increased levels of β-amyloid in 5XFAD / Neu1 −/− animals ( Fig. 5c,d ). Histological analyses of brain sections revealed higher levels of APP in the 5XFAD / Neu1 −/− subiculum when compared with the levels in the same region of the 5XFAD ( Fig. 5e ). Hence, deficiency or downregulation of NEU1 may represent a risk factor for the development of AD. 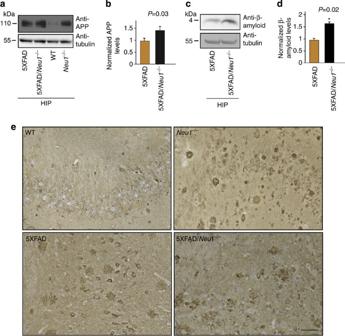Figure 5: NEU1 loss-of-function in a model of AD accelerates β-amyloid production. (a,c) APP and β-amyloid levels, respectively, were analysed in hippocampal lysates from 5XFAD, 5XFAD/Neu1−/−andNeu1−/−hippocampi. (b,d) Quantification ofaandc; the normalized levels of APP and β-amyloid were calculated by densitometric analysis of single bands on immunoblots probed with anti-APP or β-amyloid antibodies, and anti-tubulin in 5XFAD and in 5XFAD-Neu1−/−samples. Anti-tubulin antibody was used as loading controls; asterisks on graphic bars indicate statistically significant results, as determined by the Student’st-test. Data are represented as the mean±s.d. (error bars);n=3 (e) Representative pictures of full-length APP staining in WT, 5XFAD, 5XFAD/Neu1−/−andNeu1−/−hippocampal regions (5XFAD, 5XFAD/Neu1−/−mice were 3 months of age, WT andNeu1−/−mice were 5 months of age; N-terminal antibody against APP). Scale bar, 20 μm. Figure 5: NEU1 loss-of-function in a model of AD accelerates β-amyloid production. ( a , c ) APP and β-amyloid levels, respectively, were analysed in hippocampal lysates from 5XFAD, 5XFAD/ Neu1 −/− and Neu1 −/− hippocampi. ( b , d ) Quantification of a and c ; the normalized levels of APP and β-amyloid were calculated by densitometric analysis of single bands on immunoblots probed with anti-APP or β-amyloid antibodies, and anti-tubulin in 5XFAD and in 5XFAD- Neu1 −/− samples. Anti-tubulin antibody was used as loading controls; asterisks on graphic bars indicate statistically significant results, as determined by the Student’s t- test. Data are represented as the mean±s.d. (error bars); n =3 ( e ) Representative pictures of full-length APP staining in WT, 5XFAD, 5XFAD/ Neu1 −/− and Neu1 −/− hippocampal regions (5XFAD, 5XFAD/ Neu1 −/− mice were 3 months of age, WT and Neu1 −/− mice were 5 months of age; N-terminal antibody against APP). Scale bar, 20 μm. Full size image NEU1 upregulation reverses AD pathology in 5XFAD mice We next tested whether augmenting Neu1 activity in the 5XFAD model would revert or delay the amyloidogenic process. To generate high levels of Neu1 activity in the brain, we used an admixture of adeno-associated viruses (AAVs) expressing human NEU1 and its auxiliary chaperone PPCA [30] , [50] . This vector combination produced the highest NEU1 activity when transduced into Neuro2a neuroblastoma cell lines ( Supplementary Fig. S7a ). The AAV- PPCA /AAV- NEU1 mixture was stereotactically injected unilaterally into the hippocampal region of 4- to 6-month-old 5XFAD mice. Four weeks after injection, immunohistochemical analyses of brain sections revealed a remarkable overall reduction of plaque burden in the hippocampal region of the AAV-injected mice compared with that of 5XFAD mice injected only with carrier solution ( Fig. 6a,b ). This was accompanied by high levels of expression of NEU1 and PPCA in the same region of the AAV-treated mice ( Supplementary Fig. S7b,c ). We also quantified the number of amyloid plaques in serial sections of the subiculum from four AAV-injected animals and found that the surface occupied by the plaques was reduced by 44.3±6.2% in these mice, compared with the same area in the carrier solution-injected mice ( Fig. 6c ). Finally, boosting the activity of NEU1 in the hippocampal area of the AAV-injected 5XFAD had a direct effect on the levels of APP ( Fig. 6d–f ) and β-amyloid ( Fig. 6g,h ), which were substantially reduced. Collectively, these results put forward the idea that NEU1 could be an effective therapeutic agent for AD. 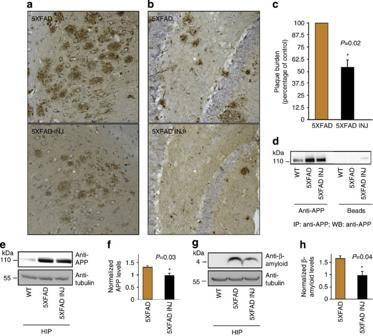Figure 6: NEU1 upregulation in 5XFAD reduces β-amyloid and plaques development. (a,b) Injection of an AAV containing humanNEU1andPPCAin the hippocampus of 4- and 6-month-old 5XFAD animals, respectively, (5XFAD INJ) reduced the number of amyloid plaques compared with that seen in 5XFAD animals injected only with carrier solution. Plaques were identified by 4G8 immunostaining (brown). (a) Scale bar, 20 μm. (b) Scale bar, 10 μm. (c) Reduction of amyloid plaques in 5XFAD INJ, as determined by quantification of 4G8 immunostaining (mean±s.d.;n=4). (d,e) NEU1 overexpression in the 5XFAD INJ mice reduces APP as demonstrated by immunoprecipitation (d) and immunoblotting (e) analyses. (f) Quantification ofe. (g) Reduction of β-amyloid levels in hippocampal lysates from 5XFAD INJ mice. (h) Quantification ofg. The 5XFAD/5XFAD INJ ratio was calculated by densitometric analysis of single bands on immunoblots probed with anti-APP or -β-amyloid antibodies and anti-tubulin in 5XFAD and in 5XFAD INJ hippocampal lysates. Asterisks on graphic bars indicate statistically significant results, as determined by the Student’st-test. Data are represented as the mean±s.d. (error bars);n>3. Figure 6: NEU1 upregulation in 5XFAD reduces β-amyloid and plaques development. ( a , b ) Injection of an AAV containing human NEU1 and PPCA in the hippocampus of 4- and 6-month-old 5XFAD animals, respectively, (5XFAD INJ) reduced the number of amyloid plaques compared with that seen in 5XFAD animals injected only with carrier solution. Plaques were identified by 4G8 immunostaining (brown). ( a ) Scale bar, 20 μm. ( b ) Scale bar, 10 μm. ( c ) Reduction of amyloid plaques in 5XFAD INJ, as determined by quantification of 4G8 immunostaining (mean±s.d. ; n =4). ( d , e ) NEU1 overexpression in the 5XFAD INJ mice reduces APP as demonstrated by immunoprecipitation ( d ) and immunoblotting ( e ) analyses. ( f ) Quantification of e . ( g ) Reduction of β-amyloid levels in hippocampal lysates from 5XFAD INJ mice. ( h ) Quantification of g . The 5XFAD/5XFAD INJ ratio was calculated by densitometric analysis of single bands on immunoblots probed with anti-APP or -β-amyloid antibodies and anti-tubulin in 5XFAD and in 5XFAD INJ hippocampal lysates. Asterisks on graphic bars indicate statistically significant results, as determined by the Student’s t- test. Data are represented as the mean±s.d. (error bars); n >3. Full size image The trafficking and deposition of progressively accumulating toxic proteins by diseased neurons is a crucial but poorly understood issue in the field of neurodegenerative diseases. Autophagy and lysosomal mechanisms of degradation have been rapidly emerging areas of interest in this regard [51] , [52] . The notion that neurons could release abnormal proteins by lysosomal exocytosis has been postulated but, until now, there was no evidence for such a process. Moreover, the concept that β-amyloid deposited extracellularly in the AD brain could originate from intraneuronal production in the endosomal–lysosomal compartment [23] , [47] has hinted on exocytic processes as likely to be additional mechanisms for the release of Aβ. Most importantly, the oligomerization/aggregation of Aβ is favoured by an acidic environment [6] , which further indicates that initial oligomerization within the acidic endosomes/lysosomes coupled to a regulated lysosomal release mechanism could be critical in the Aβ toxic life cycle. In this study, we identify a central role for NEU1 in regulating both the fate of APP by cleaving its sialic acids and the extracellular release of Aβ by lysosomal exocytosis ( Fig. 7 ). Our data on APP sialic acid content agree with earlier studies that found a positive correlation between increased APP sialylation by overexpression of the α-2,6-sialyltransferase ST6Gal-I and the extracellular release of its metabolites, promoting the secretion of amyloid-β peptides [48] . This implies that either the biosynthetic or the catabolic control of the sialic acids on APP affects its β-amyloidogenic processing. We propose that in the absence of NEU1, the oversialylation of APP may change its half-life and lead to accumulation of it and/or its metabolites in the endosomal–lysosomal compartment. This accumulated APP would then be more prone to β-amyloidogenic cleavage, resulting in accelerated production of neurotoxic APP end products by the neuronal β-secretase. In this regard, it is noteworthy that BACE1 was shown to reside in the lumen of an acidic intracellular compartment and to function at acidic pH [53] . Altogether, our findings favour a lysosomal control over the levels of APP and its proteolytic cleavage, which we believe are directly relevant to the pathogenesis of AD. 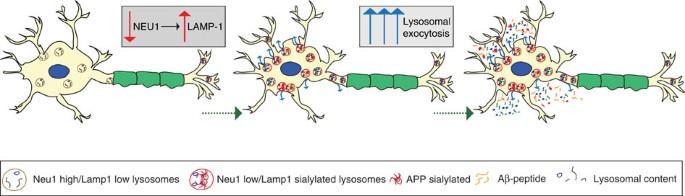Figure 7: Schematic model. In the absence of Neu1, oversialylated APP is abnormally processed in lysosomes and the generated Aβ−peptide is released in the extracellular space via excessive lysosomal exocytosis. Figure 7: Schematic model. In the absence of Neu1, oversialylated APP is abnormally processed in lysosomes and the generated Aβ−peptide is released in the extracellular space via excessive lysosomal exocytosis. Full size image It has been postulated that proteolytically generated Aβ peptides may engage in a prion-like mechanism of spreading and be transmitted from cell to cell [54] or deposited extracellularly by processes that involve microvesicles or cellular nanotubes [13] . We now provide evidence that excessive lysosomal exocytosis downstream of Neu1 deficiency mediates the release of Aβ, a finding that identifies this process as a plausible mode of spreading of the toxic peptide ( Fig. 7 ). Moreover, excessive release of endolysosomal contents may create in the immediate vicinity of the PM of cells and the extracellular space, an ideal acidic microenvironment that would favour the continuous processing, aggregation and fibrillation of Aβ, ultimately resulting in plaque formation [7] , [8] , [55] . This kind of pathogenic cascade is also in agreement with a large body of work that has involved the endocytic pathway as a major contributor to AD [25] , [56] , [57] . Increased endocytosis in AD increases the delivery of substrates, including APP and its metabolites, to endolysosomes [56] . The accumulation of incompletely degraded cargoes within NEU1-deficient dysfunctional lysosomes could then contribute to further release of Aβ by lysosomal exocytosis. It is conceivable that excessive lysosomal exocytosis may be counterbalanced by further increased endocytosis to maintain PM integrity. In this scenario, endolysosomes would be engaged in a self-propagating pathogenic loop, which eventually promotes the generation of Aβ in the endolysosomal compartment and its subsequent exocytosis. Another feature that can be indicative of deregulated lysosomal exocytosis is the increased expression of the NEU1 substrate LAMP1. This protein is present in an oversialylated state in neurons of the Neu1 −/− model. Consistent with this finding, LAMP1 has been found to be upregulated both in AD patients and animal models of the disease, and shown to increase in amounts with disease progression [23] , [58] , [59] , reiterating the notion that lysosomes are actively engaged in AD pathogenesis. Furthermore, if NEU1 downregulation will be proven in AD brain specimens, the relative levels of NEU1 and LAMP1 may be suggestive of excessive lysosomal exocytosis. Only 1–5% of AD cases are familial AD (FAD), that is, linked to known genetic mutations, and usually develop an early-onset form of the disease. The vast majority of the patients contracts the so-called sporadic AD of still unknown aetiology and mostly associated with aging [60] . Given the complexity of this disease, it is foreseeable that it may result from the interplay between deterministic or risk genes, and epigenetic and environmental factors. So far, the strongest genetic risk factor found in sporadic AD patients is apolipoprotein E, genotype ε4, which is thought to increase the rate of aggregation and decrease the clearance of Aβ [61] , albeit by still not fully understood mechanisms. We now propose NEU1 as a potential, novel risk factor in hastening the progression of AD. We show that Neu1 deficiency have an additive effect when combined with familial AD mutations in the 5XFAD transgenic model in accelerating β-amyloid formation. We are tempted to speculate that genetic or epigenetic downregulation of NEU1 may exacerbate the development and progression of AD in some of the sporadic cases, although further studies are required to validate this hypothesis. The need for developing effective treatments for AD is becoming urgent given the projected number of people worldwide, who will present with the disease within the next four decades [3] , [60] . Despite tremendous scientific effort, at the moment the available drugs used in AD patients have had only modest and transient effects, which exclude their curative potential. Recently, new therapeutic strategies have proven to be effective in clearing extracellular β-amyloid deposition in AD mouse models [62] , but it is still uncertain whether these approaches may be effective in addressing the intracellular pathobiology, including lysosomal clearance deficits and intraneuronal Aβ toxicity, which may be critical for neurodegeneration. As demonstrated in this study, AAV-mediated gene therapy could be a suitable therapeutic strategy for AD, because it has been successfully applied in clinical trials and preclinical studies [50] , [63] . On the basis of our findings that increasing Neu1 activity in the brain of the 5XFAD mice reduces their β-amyloid plaque burden, we propose that upregulation of NEU1 could be exploited as a novel therapeutic strategy to halt or revert disease pathogenesis. Animal models All procedures in mice were performed according to animal protocols approved by the St Jude Children’s Research Hospital Institutional Animal Care and Use Committee and NIH guidelines. Neu1 −/− and WT mice were bred into the FVB/NJ and C57BL/6 genetic backgrounds. 5XFAD transgenic mice were obtained from the Jackson Laboratory. Enzymatic activities NEU1 and β-hex catalytic activities were measured against synthetic substrates 2′-(4-methylumbelliferyl)-α- D -N-acetylneuraminic acid, sodium salt and 4MU-N-acetyl-β- D -glucosaminide as reported previously [31] . Briefly, cells were collected and lysed in water for both assays. To measure NEU1 enzymatic activity, 5 μl of homogenate was incubated with 5 μl of 2′-(4-methylumbelliferyl)-α- D -N-acetylneuraminic acid, sodium salt in triplicate in 96-well plates for 1 h at 37 °C. To assay β-hex activity, 10 μl of homogenate was incubated with 10 μl of 4MU-N-acetyl-β- D -glucosaminide. To stop enzyme reactions, 200 μl of 0.5 M carbonate buffer, pH 10.7, was added to all wells. The fluorescence was measured on a plate reader (EX-355, EM-460). The net fluorescence values were compared with those of the linear 4MU standard curve and were used to calculate the specific enzyme activities. Activities were calculated as nanomoles of substrate converted per hour per milligrams of protein (nmol h −1 mg −1 ). Acid phosphatase activity was assayed with the help of the acid phosphatase assay kit from Sigma, according to the manufacturer’s instruction. Media from different cells was collected and centrifuged at 11,000 g for 5 min. Spun-down medium was then applied onto a G50 Sephadex column packed in an acidic buffer before performing enzymatic assays. Enzyme-linked immunosorbent assay of Aβ1-42 The amount of mouse A β 1-42 and human A β 1-42 in the cell culture media and in the cerebrospinal fluid was determined by using mouse and human A β 42 enzyme-linked immunosorbent assay kit (Invitrogen) following manufacturer’s instructions. Mouse A β and human A β levels were normalized to total protein levels and total cell number, respectively. Antibodies and reagents We used the following commercial antibodies: anti-LAMP1 (Sigma; 1:500), anti-α/β-tubulin (Cell Signaling; 1:1,000), anti-GFAP (DAKO; 1:1,000), anti-β-III tubulin (TUJ1. Covance; 1:500), anti-APP (22C11, Millipore; 1:500), anti-APP/Aβ (4G8, Covance; 1:500), anti-Aβ (12F4, Covance; 1:500), pan-anti-Aβ (Covance; 1:50), anti-ubiquitin (DAKO; 1:1,000) and anti-neurofilaments (DAKO; 1:1,000). Anti Neu1 and anti-cathepsin A (PPCA) antibodies were generated in our laboratory. The anti-C1/6.1 antibody (anti-CTF) was provided by Dr Nixon. CY3- and horeseradish peroxidase-conjugated secondary antibodies were purchased from Jackson ImmunoResearch Laboratory (West Grove, PA); 488- and 594- conjugated secondary antibodies were from Molecular probes. Sanbucus nigra lectin was obtained from Vector Laboratories (Burlingame, CA) and used at 1:500 dilution. Lysotracker Red DND-99 was obtained from Invitrogen and was applied as per the manufacturer’s instructions. TAMRA-Aβ1-42 was purchased from Anaspec. Cell culture For neurospheres cultures, hippocampi were dissected from brains of P3 to P6 Neu1 −/−Arf , WT Arf and β-gal −/− mice (mixed sex) and dissociated into a single-cell suspension by 5 min incubation in TrypLE Express (Invitrogen) and triturated with glass pipettes. For immunofluorescence (IF) analysis, neurospheres were transferred onto glass coverslips, coated sequentially with poly- L -ornithine (10 μg ml −1 ; Sigma) and laminin (5 μg ml −1 ; Invitrogen). After an additional 48 h, attached neurospheres were fixed in PBS containing 4% paraformaldehyde, washed and processed for immunocytochemical analysis. Images were analysed with confocal laser scanning microscope (Leica, TCS-NTSP). Astrocytes were isolates from P1-3 postnatal animals and dissociated into a single-cell suspension by 5 min incubation in 2.5% trypsin (Invitrogen) and 1% (wt/vol) DNase (Invitrogen), and triturated with glass pipettes. Single cells were resuspended in growth medium containing MEM (Invitrogen) supplemented with 5% fetal bovine serum (Sigma) and 5% horse serum (Invitrogen). For cell-uptake experiments, neurospheres were dissociated an attached on laminin/poly- L- ornithine-coated slides and incubated with 250 nM TAMRA-Aβ1-42. After incubation with TAMRA-Aβ1-42, neurospheres were washed to remove the compound present in the culture medium. After 24 h of recovery time, medium was collected in a plate that was excited at 535 nm as a measure of TAMRA-Aβ1-42 exocytosed. Neuro2a, a mouse neuroblastoma cell line, was kindly provided by Dr Nixon. This line was used as in vitro model system to test NEU1 activity after AAV particle transduction. These cells were maintained in DMEM media (Invitrogen) supplemented with Glutamax (Sigma), penicillin and streptomycin (Invitrogen), and 10% cosmic calf serum (Hyclone). Hippocampal neurospheres were differentiated into neurons using a recombinant basic fibroblast growth factor stimulation method, which promotes the proliferation of neuronal progenitors before differentiation [44] , following a procedure outlined by Stemcell Technologies. Briefly, 25,000 dissociated neurospheres cells were plated onto poly- D -lysine (100 μg ml −1 ; Invitrogen)-coated slides in DMEF:F12 plus N2 supplement (Invitrogen), containing recombinant basic fibroblast growth factor to a final concentration of 20 ng ml −1 without serum. The next day, cells were washed and neuronal basal medium plus SM1 supplement (Stemcell Technologies) was added. Differentiated cells were analysed by IF with neuronal and glial markers. Calcimycin treatment and lysosomal exocytosis inhibition To induce fusion of docked lysosomes to the PM and extracellular release of their luminal contents, neurospheres were dissociated, counted and plated. They were incubated for 30 min in medium containing 10 μM Calcimycin A23187 (Sigma) in the presence of 1.2 mM CaCl 2 . In some instances, to inhibit lysosomal exocytosis, cells were washed with Ca 2+ -free PBS and further maintained in Ca 2+ -free medium containing 10 mM EGTA, before the addition of calcimycin and CaCl 2 . Immunoblotting Hippocampi were homogenized with a buffer containing: 1% Nonidet P-40, 0.1% SDS, 50 mM Tris, pH 8.0, 50 mM NaCl, 0.05% deoxycholate, and protease inhibitor. Lysosomes were purified from hippocampi of WT and Neu1 −/− mice using the Lysosome Isolation Kit (Sigma) following the manufacturer’s protocol, with slight modifications. In brief, hippocampi from four WT and Neu1 −/− mice were homogenized in four volumes of 1 × extraction buffer in a glass Dounce homogenizer. The nuclei were removed by centrifugation at 1,000 g for 10 min. The post-nuclear supernatant was centrifuged at 20,000 g for 20 min and the resulting pellet, containing the crude LF, was resuspended in a minimal volume of 1 × extraction buffer and loaded onto a Optiprep density gradient and centrifuged at 150,000 g for 4 h. Fractions (0.5 ml) were collected starting from the top of the gradient. Each fraction was assayed for protein concentration and acid phosphatase activity (Sigma). Protein concentrations were determined using the BCA assay (Pierce Biotechnology). Proteins were separated by SDS–PAGE (4–12%, 4–20%, 12% Bis-Tris gel, Invitrogen) under reducing conditions and transferred to a polyvinylidene difluoride membrane (Millipore). Membranes were incubated for 1 h in blocking buffer and subsequently probed with the specific antibody overnight. Immunoblots were developed by using Enhanced Chemiluminescence Kit (Perkin Elmer Life Sciences) or SuperSignal West Femto Chemiluminescent Substrate (Pierce). For amyloid detection, before the blocking step, membranes were incubated in 0.2% glutaraldehyde in PBS for 45 min. For immunoprecipitation analyses, hippocampal extracts (500 μg) were diluted in 250 μl PBS/0.2% BSA with antibodies (2.5 μg anti-APP, 4G8 or 22C11) overnight at 4 °C on a rocking platform. Samples were incubated for an additional hour after the addition of BSA (2%) blocked Protein G beads (Invitrogen). The beads were washed three times in PBS and proteins were eluted with sample loading buffer before immunoblot (4–12% Bis-Tris gel, Invitrogen). Proteins then transferred onto polyvinylidene difluoride membranes were probed with an anti-APP antibody or biotynilated S. nigra lectin. Full gel scans can be found in Supplementary Figs S8–S11 . Methoxy-XO4 in vivo injections For in-vivo imaging studies, WT and Neu1 −/− mice ( n =3) were injected intraperitoneally with 10 mg kg −1 Methoxy-X04 (ref. 45 ). Mice were anaesthetized and perfused with PBS 24 h after the injection. The brains were collected, sliced at 200 μm and imaged. Three-dimensional renderings of Methoxy-XO4-labelled amyloid were created from z -stack acquisitions using Imaris 6.0 software. Immunohistochemistry and IF analyses Mouse brains were collected after PBS perfusion and fixed with 4% paraformaldehyde for 12 h at 4 °C. Brain tissues were incubated overnight in 20% sucrose at 4 °C. Finally, tissues were embedded in tissue-freezing medium (Triangle Biomedical Sciences, Inc.) and snapfrozen in liquid nitrogen. Immunohistochemistry (IHC) and IF analyses were performed on 10-μm-thick serial cryosections or paraffin sections. For IHC analysis, after blocking (0.1% BSA, 0.5% Tween-20 and 10% normal serum), sections were incubated overnight at room temperature with the specific antibody diluted in blocking buffer. The sections were washed and incubated with biotinylated secondary antibody (Jackson ImmunoResearch Laboratory) for 1 h. Endogenous peroxidase was removed by incubating the sections with 0.1% hydrogen peroxidase for 30 min. Antibody detection was performed using the ABC Kit and diaminobenzidine substrate (Vector Laboratories) and sections were counterstained with haematoxylin according to standard method. For IHC analysis with 4G8 or Aβ42 antibodies, tissue sections were pretreated with formic acid (70%) before the blocking step. For IF, after blocking with 0.1% BSA, 0.2% saponin and 10% normal serum, the specific antibody diluted in blocking buffer was applied overnight at room temperature. The sections were washed and incubated with fluorescent secondary antibody (Jackson ImmunoResearch Laboratory and Molecular probes, Invitrogen) for 1 h. Stained sections were mounted with prolong Gold with 4',6-diamidino-2-phenylindole (Invitrogen). For lysotracker fluorescence microscopy, dissociated neurospheres were seeded on laminin/poly- L -ornithine slides and incubated for 30 min at 37 °C in medium containing 200-nM Lysotracker (DND-99, Invitrogen). TIRFM of live lysotracker-labelled neurospheres was performed with a Marianas imaging system (Intelligent Imaging Innovations/3i) consisting of a Carl Zeiss 200M motorized inverted microscope and TIRF illuminator (Carl Zeiss MicroImaging) and a DPSS 561 nm laser (Cobolt). Images were acquired with a Zeiss Alpha Plan-Fluar 100 × 1.45 numerical aperture objective on a CoolSNAP HQ 2 charge-coupled device camera (Photometrics), using SlideBook 4.2 software (3i). Confocal microscopy on lysotracker-stained live cells and IF analysis on brain sections were performed with an inverted microscope equipped with a C1Si confocal system. Lysosomes and TAMRA-Aβ1-42 were identified as objects and counted in more than ten TIRFM images. Electron microscopy For the ultrastructural studies, hippocampi were fixed and embedded using standard protocols and sections (600–900 Å) were stained in grids and visualized using a JEOL-JEM 1200EX II Electron Microscope and a Gatan 782 Digital Camera. Vector production The scAAV2/8-CMV-PPCA (PPCA) and scAAV2/8-CMV-NEU1 (NEU1) constructs contain a cytomegalovirus ( CMV ) promoter, which ensures expression of the 1.44-kb human PPCA complementary DNA and 1.247-kb human NEU1 cDNA. The scAAV vector particles were made in the Children’s Good Manufacturing Practice, LLC facility on the St Jude campus. scAAV2/8-CMV-PPCA and scAAV2/8-CMV-NEU1 vector genome titres were determined by quantitative PCR and/or direct loading and electrophoresis of detergent-treated vector particles on native agarose gels, staining with fluorescent dye, quantification of signal relative to known mass standards. AAV transduction in vitro and in vivo Neuro2a cells were transduced with 5,000 genome-containing (GC) particles of scAAV2/8-CMV-PPCA and 1700 GC of scAAV2/8-CMV-NEU1, either alone or in combination in 500 μl of Optimem (Invitrogen). After 90 min incubation with vectors, complete culture medium was added to the cells that were grown for 2 days. Cell pellets from not-transduced and transduced cells were used for NEU1 enzymatic activity assays. For the transduction in vivo , 5XFAD mice (4–6 months old; n =2 for each age) were anaesthetized and placed into a Kopf stereotaxic device. Injections were done unilaterally into the left hippocampus. Injections were performed with a 10-μl Hamilton syringe fitted with a glass micropipette. 10 μl of virus (mixture of PPCA virus, 2 × 10 11 GC and NEU1 virus, 0.7 × 10 11 GC) or 10 μl of carrier solution per brain. For all the brain injections, the needle was left in place for 5 min before withdrawal from the brain. Four weeks after the injection, mice were killed and the brains were processed for amyloid (4G8 antibody), NEU1 and PPCA stainings. Amyloid counts Quantification of β-amyloid plaques was carried out on IHC images captured from sections stained with anti-APP/Aβ antibody (4G8 antibody). IHC images were first transformed to monochrome and inverted to make amyloid plaques bright areas. Sections of each mouse brain were imaged, and the areas and densities of the plaques present in the subiculum dentate gyrus areas were measured using NIS-Elements 3.22.11 Software (Nikon Instruments, Inc., Melville, NY). An intensity threshold level was established to discriminate between plaque immunostating and background labelling. The threshold for detection was held constant throughout the image quantification. An object of interest was defined by its surface and its brightness. Statistical analysis Data are expressed as mean±s.d. and were evaluated using the Student’s t -test for unpaired samples. P -values<0.05 were considered statistically significant. How to cite this article: Annunziata, I. et al. Lysosomal NEU1 deficiency affects amyloid precursor protein levels and amyloid-β secretion via deregulated lysosomal exocytosis. Nat. Commun. 4:2734 doi: 10.1038/ncomms3734 (2013).